High-efficiency translational bypassing of non-coding nucleotides specified by mRNA structure and nascent peptide The gene product 60 (gp60) of bacteriophage T4 is synthesized as a single polypeptide chain from a discontinuous reading frame as a result of bypassing of a non-coding mRNA region of 50 nucleotides by the ribosome. To identify the minimum set of signals required for bypassing, we recapitulated efficient translational bypassing in an in vitro reconstituted translation system from Escherichia coli . We find that the signals, which promote efficient and accurate bypassing, are specified by the gene 60 mRNA sequence. Systematic analysis of the mRNA suggests unexpected contributions of sequences upstream and downstream of the non-coding gap region as well as of the nascent peptide. During bypassing, ribosomes glide forward on the mRNA track in a processive way. Gliding may have a role not only for gp60 synthesis, but also during regular mRNA translation for reading frame selection during initiation or tRNA translocation during elongation. The ribosome is a molecular machine that translates the nucleotide (nt) sequence of the mRNA into the co-linear amino-acid sequence of a protein. In general, the co-linearity is maintained by sophisticated mechanisms that ensure that the ribosome moves on the mRNA track in a stepwise manner, by precisely one codon at a time, and each codon in the open reading frame (ORF) is translated into an amino acid in the protein. There are only a few cases known where the amino-acid sequence of a protein is not co-linear with the mRNA. Until recently, one well-documented case for a programmed non-co-linear mRNA translation was provided by the gene 60 mRNA of bacteriophage T4 that codes for a subunit of a DNA topoisomerase (gene product 60, gp60). Recent evidence suggests that bypassing phenomena may be more common than assumed so far; for example, the prevalence of ribosome bypassing was demonstrated in mitochondria of the yeast Magnusiomyces capitatus [1] , and there are further strong candidates for novel cases of translational bypassing [2] . During translation of gp60 mRNA, the ribosome produces a single polypeptide chain from a discontinuous reading frame [3] , [4] . The interrupted ORF is unique to the T4 genome and is caused by the disruption of gene 39 , which encodes the DNA topoisomerase subunit in other T-even bacteriophages [5] , by the insertion of a mobile DNA element [6] . The mobile element splits gene 39 into a sequence coding for the N-terminal part of gp39 and the newly formed gene 60 , which codes for the C-terminal portion of the topoisomerase. One consequence of the mobile element insertion is the addition within the gene 60 coding sequence of a 50-base pair foreign sequence [6] , which is copied into the gene 60 mRNA. The non-coding sequence is not spliced but is skipped during translation [3] , [4] . The ribosome translates the first 46 codons of gene 60 mRNA up to the glycine codon GGA followed by a stop codon UAG ( Fig. 1a ). However, instead of terminating translation at the stop codon, peptidyl-tRNA 2 Gly disengages from pairing with the GGA codon 5′ adjacent to the coding gap, is retained within the ribosome as it slides over the 50-nt non-coding gap and re-pairs to mRNA at the triplet, also GGA, 5′ adjacent to the coding resumption site [7] . Disengagement is referred to as occurring at the ‘take-off’ codon with re-pairing to mRNA being at the ‘landing site’ codon, which is complementary to the anticodon. The take-off codon is 5′ adjacent to UAG and both are near the top of a stem loop (SL), the ‘take-off SL’ that is critical for bypassing [4] , [7] , [8] , [9] , [10] . The analysis of the mRNA structure suggested that the gap region is structurally autonomous from the upstream and downstream coding regions [10] , consistent with the evolutionary origin of the gap from a mobile element [6] . The presence of the take-off GGA and the matching landing codons, the UAG stop codon next to the take-off GGA and the SL structure in the 5′ gap are essential for bypassing. Also the identity of peptidyl-tRNA 2 Gly that remains bound to the ribosome during bypassing is crucial, as other tRNAs support bypassing to different, but generally substantially lesser extent [11] , [12] . A short potential Shine-Dalgarno (SD)-like GAG sequence 6 nt 5′ of the GGA landing site contributes to the precision of landing [9] . Furthermore, part of the nascent peptide is important for bypassing efficiency [4] , with preliminary evidence pointing to the significance of a KKYK motif [13] . Finally, genetic experiments with mutants containing an enlarged SL indicated an important role of ribosomal protein L9 (ref. 14 ), which subsequently was shown to have a role in normally restraining forward mRNA slippage [11] . These diverse stimulatory elements are likely to provide a complex regulatory network of physical interactions and, presumably, kinetic effects that influence bypassing [15] . 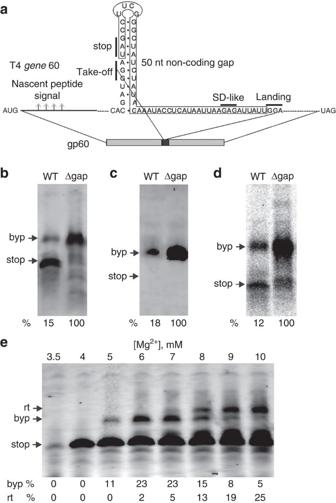Figure 1: Peptide products upon translation ofgene 60mRNAin vitro. (a) Schematic of phage T4gene 60mRNA and the respective full-length peptide product gp60. The take-off and landing codons (GGA), the stop codon (UAG) and the potential SD-like sequence (GAG) preceding the landing codon are indicated; the putative enhancing signals of the nascent peptide are shown by arrows. The non-coding 50-nt gap encompasses the sequence between the UAG stop codon and the codon preceding the landing GGA. The resulting product, the topoisomerase subunit gp60, is composed of the N-terminal part (grey area) corresponding to the mRNA sequence upstream of the internal stop codon, a Gly encoded by the take-off and landing site codons (black square), and the C-terminal part (grey area) encoded by the downstream mRNA sequence; the N- and C- terminal parts are not shown to scale. (b–d) Products of thein-vitrotranslation of a 455-nt-long fragment ofgene 60mRNA. Proteins were separated by SDS–polyacrylamide gel electrophoresis and detected using the fluorescence of the N-terminal BPY-Met (b); the C-terminal LUMIO-tag (c); or radioactivity of [14C]Leu in peptides (d); note that there is a single Leu residue in the N-terminal part of pg60 preceding the Gly at position 46, compared with five Leu residues in the full-length product. WT, the construct containing the gap region. Δgap, the construct in which the gap region was deleted and the N- and C-terminal parts of gp60 are fused in frame. (e) Effect of Mg2+concentration on the efficiency and fidelity of bypassing. stop, the N-terminal 46 amino acids long peptide terminated at the UAG stop codon immediately following the take-off GGA; byp, the protein product of bypassing (88 amino acids); read-through (rt), the protein product synthesized when an amino acid is incorporated in place of stop codons (105 amino acids). For each translation experiments, two independent repeats were carried out (n=2). Figure 1: Peptide products upon translation of gene 60 mRNA in vitro . ( a ) Schematic of phage T4 gene 60 mRNA and the respective full-length peptide product gp60. The take-off and landing codons (GGA), the stop codon (UAG) and the potential SD-like sequence (GAG) preceding the landing codon are indicated; the putative enhancing signals of the nascent peptide are shown by arrows. The non-coding 50-nt gap encompasses the sequence between the UAG stop codon and the codon preceding the landing GGA. The resulting product, the topoisomerase subunit gp60, is composed of the N-terminal part (grey area) corresponding to the mRNA sequence upstream of the internal stop codon, a Gly encoded by the take-off and landing site codons (black square), and the C-terminal part (grey area) encoded by the downstream mRNA sequence; the N- and C- terminal parts are not shown to scale. ( b – d ) Products of the in-vitro translation of a 455-nt-long fragment of gene 60 mRNA. Proteins were separated by SDS–polyacrylamide gel electrophoresis and detected using the fluorescence of the N-terminal BPY-Met ( b ); the C-terminal LUMIO-tag ( c ); or radioactivity of [ 14 C]Leu in peptides ( d ); note that there is a single Leu residue in the N-terminal part of pg60 preceding the Gly at position 46, compared with five Leu residues in the full-length product. WT, the construct containing the gap region. Δgap, the construct in which the gap region was deleted and the N- and C-terminal parts of gp60 are fused in frame. ( e ) Effect of Mg 2+ concentration on the efficiency and fidelity of bypassing. stop, the N-terminal 46 amino acids long peptide terminated at the UAG stop codon immediately following the take-off GGA; byp, the protein product of bypassing (88 amino acids); read-through (rt), the protein product synthesized when an amino acid is incorporated in place of stop codons (105 amino acids). For each translation experiments, two independent repeats were carried out ( n =2). Full size image The exact mechanism of how the ribosome traverses the gap sequence and why it lands at the particular landing codon is not known. Important unresolved questions are how and why ribosomes can override the regular co-linearity of mRNA and protein sequence, whether it requires auxiliary factors for bypassing, and how such an unusual recoding event relates to the normal function of the ribosome. To address these questions, we set out to investigate bypassing in vitro in a fully reconstituted translation system consisting of purified, biochemically defined components only. Here we recapitulate efficient and accurate bypassing in a minimum translation system in the absence of any auxiliary factors, indicating that the signals crucial for bypassing are contained in the gene 60 mRNA sequence itself. Our analysis suggests unexpected layers of signals specified in the mRNA secondary structure and in the sequence of the nascent peptide, and provides a quantitative model that describes translational bypassing as processive ribosome gliding over the mRNA track. Efficient and accurate bypassing in vitro Bacteriophage T4 gene 60 mRNA was translated in a reconstituted synchronized translation system containing 70S initiation complexes, elongation factors (EF-Tu, EF-G) and purified aminoacyl-tRNAs from E. coli . To visualize translation products, initiation complexes were prepared using fluorescence-labelled Bodipy FL-Met-tRNA fMet (Bpy-Met-tRNA fMet ; Fig. 1b ). Translation of the gene 60 mRNA comprising 322 nt of the wild-type (WT) coding sequence gave rise to two distinct peptide bands (approximately 5 and 11 kDa). The shorter product corresponded to the gp60 sequence up to the take-off Gly codon (denoted as ‘stop’). The full-length product (bypassing product, denoted as ‘byp’) resulted from the translation of two non-contiguous ORFs. The size of the byp was validated using a construct in which the two reading frames were fused by omission of the bypassing gap (Δgap). The correct reading frame of the byp was verified using the C-terminal Lumio-tag introduced in-frame with gp60 ( Fig. 1c ). The efficiency of translation bypassing was quantified using the fluorescence of Bpy or Lumio, and by autoradiography based on [ 14 C]Leu incorporated into the WT or Δgap products ( Fig. 1d ). According to the three reporters ( Fig. 1b–d ), and comparing with the WT control in the experiments described below ( Fig. 1e and 4b, etc. ), bypassing was observed on about 15–25% of translating ribosomes, comparable to bypassing efficiencies measured in vivo . These results suggest that the synthesis of gp60 in a well-defined reconstituted in vitro translation system results in efficient bypassing, which does not require any additional auxiliary factors. Thus, the major signals required for translational bypassing must reside in the mRNA itself. Both efficiency and fidelity of bypassing were further tested by varying the Mg 2+ concentration ( Fig. 1e ). The Mg 2+ concentration is crucial for speed and fidelity of decoding [16] ; however, its effect on recoding events, such as bypassing, is not known. At low Mg 2+ concentration, the gene 60 mRNA was translated up to the stop codon at the beginning of the gap, but the full-length byp was not formed (we have added 3.5–4.0 mM Mg 2+ , corresponding to about 1.0–1.5 mM of free Mg 2+ , taking into account the Mg 2+ bound to GTP and phosphoenol pyruvate present in the reaction mixture [16] ; see Methods). At higher concentrations of Mg 2+ (5–7 mM added), the byp was formed (23%). When the Mg 2+ concentration was increased further, additional translation products appeared, including the product of the stop-codon read-through (upper band, ‘rt’), suggesting that the fidelity of decoding was compromised. Efficiency and fidelity of translation and bypassing can be additionally tuned by polyamines ( Supplementary Fig. 1 ). Generally, at low Mg 2+ concentrations, the addition of spermidine and putrescine facilitated bypassing; however, the read-through efficiency was increased as well. Spermine induced significant misreading even at low concentrations. Given the complex interplay between Mg 2+ and polyamines and the narrow optimum in polyamine concentrations, we chose to work without polyamines at conditions of maximum efficiency and fidelity of recoding (7 mM added Mg 2+ , which corresponds to about 4.5 mM free Mg 2+ (ref. 16 ). Role of the nascent peptide Having established conditions for efficient bypassing, we next examined the roles of distinct regions of the gene 60 mRNA and of the nascent peptide. To study the effect of the N-terminal part of the nascent peptide, we deleted the mRNA sequence coding for amino acids 1–13 (Nascent Peptide construct 1, NP1; Fig. 2a ); the deletion reduced the bypassing efficiency by >50%, in agreement with an earlier report [4] . In order to distinguish effects potentially caused by alterations in the mRNA structure from those of amino-acid replacements, we introduced non-synonymous mutations (NP2) or synonymous replacements by other frequent codons (NP3). Both variants supported efficient bypassing, suggesting that the amino-acid composition of the N-terminal part of the nascent peptide, as well as any secondary structure of the respective mRNA region, did not affect bypassing. Together with the results of the deletion experiment, these data suggest that the contribution of the N-terminal part of gp60 may be unspecific, for example, contributing to anchoring the peptidyl moiety of peptidyl-tRNA 2 Gly during traversing the gap, when the tRNA on the ribosome is not stabilized by codon–anticodon interaction. 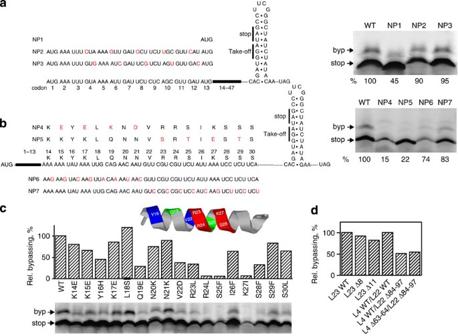Figure 2: Bypassing signals in the nascent peptide. (a) Left panel, mRNA sequence coding for the N-terminal part of gp60 (amino acids 1–13). In the mRNA construct NP1 (Nascent Peptide 1), the first 36 nucleotides are deleted. NP2 and NP3 constructs have mutations in either the 1st (NP2) or 3rd (NP3) position of codons 4, 6, 8, 10 and 12. Right panel, bypassing with NP1, NP2 and NP3 constructs, the efficiencies relative to the WT parent construct are shown below the gel. (b) Left panel, mRNA and protein sequence corresponding to the middle part of the nascent peptide (amino acids 14–30). Amino-acid replacements introduced in constructs NP4 and NP5 are shown on top. Synonymous replacements (NP6 and NP7) are shown below the WT sequence. Right panel, bypassing with mRNA constructs NP4–NP7. (c) Effect of point mutations of amino-acid residues 14–30. Relative bypassing efficiencies (upper panel) were estimated from the band intensities (lower panel); bypassing obtained with the WT construct was set to 100%. Inset, the positions of amino acids which have a significant effect on translational bypassing on an α-helix predicted by PSIPRED (http://bioinf.cs.ucl.ac.uk/psipred/). (d) Effects of mutations in ribosomal proteins L23, L22 and L4. Bypassing efficiencies were calculated relative to those measured with the isogenic WT ribosomes (n=2). Figure 2: Bypassing signals in the nascent peptide. ( a ) Left panel, mRNA sequence coding for the N-terminal part of gp60 (amino acids 1–13). In the mRNA construct NP1 (Nascent Peptide 1), the first 36 nucleotides are deleted. NP2 and NP3 constructs have mutations in either the 1st (NP2) or 3rd (NP3) position of codons 4, 6, 8, 10 and 12. Right panel, bypassing with NP1, NP2 and NP3 constructs, the efficiencies relative to the WT parent construct are shown below the gel. ( b ) Left panel, mRNA and protein sequence corresponding to the middle part of the nascent peptide (amino acids 14–30). Amino-acid replacements introduced in constructs NP4 and NP5 are shown on top. Synonymous replacements (NP6 and NP7) are shown below the WT sequence. Right panel, bypassing with mRNA constructs NP4–NP7. ( c ) Effect of point mutations of amino-acid residues 14–30. Relative bypassing efficiencies (upper panel) were estimated from the band intensities (lower panel); bypassing obtained with the WT construct was set to 100%. Inset, the positions of amino acids which have a significant effect on translational bypassing on an α-helix predicted by PSIPRED ( http://bioinf.cs.ucl.ac.uk/psipred/ ). ( d ) Effects of mutations in ribosomal proteins L23, L22 and L4. Bypassing efficiencies were calculated relative to those measured with the isogenic WT ribosomes ( n =2). Full size image Following previous reports [4] , [9] , [17] , we next tested the effect of non-synonymous (NP4 and NP5) and synonymous (NP6 and NP7) replacements introduced in codons 14–21 and 22–30 ( Fig. 2b ). Amino-acid exchanges inhibited bypassing, whereas synonymous replacements had very little effect ( Fig. 2b ), indicating that the sequence of the nascent peptide, rather than the mRNA sequence, was important. We note that alterations in the mRNA sequence resulted in decreased overall translation levels (see the stop bands in NP4 and NP6). As none of the synonymous replacements involved rare codons, the generic effect on translation probably reflects an altered mRNA secondary structure. To further identify the amino-acid positions that are critical for bypassing, we constructed mRNAs with single amino-acid replacements at each position between amino acids 14 and 30 positions ( Fig. 2b,c ). Given the length of the ribosomal peptide exit tunnel [18] , amino acids 14–30 and the following 17 amino acids of the nascent peptide up to the take-off Gly should reside within the ribosome tunnel. The mutations in the KKYK motif resulted in about 50% inhibition, mostly due to Y16, whereas substitutions of Q19, V22, R23 and S28 decreased the bypassing efficiency by 60–70%, whereas R24, S25, K27 essentially abolished bypassing. Secondary structure predictions suggest that the 14–30 region of the nascent peptide has a high propensity of helix formation with amino acids Y16, Q19, R23, R24, K27 and S28 found on the same face of the potential α-helix ( Fig. 2c , inset). The presumed α-helix may interact with the exit tunnel wall, thereby further stabilizing peptidyl-tRNA 2 Gly binding while the ribosome traverses the gap. When peptidyl-tRNA 2 Gly is formed, the length of the nascent peptide is about 20 amino acids, placing the exchanged residues in the middle part of the peptide exit tunnel, beyond the constriction formed by ribosomal proteins L4 and L22 (ref. 19) [19] . Although it is difficult to predict the exact location of the nascent peptide 14–30 region in the tunnel, we tested whether mutations of the proteins L4 and L22, as well as of ribosomal protein L23, which resides at the tunnel exit and is involved in signalling from inside the tunnel to the outside [20] , affect bypassing. Deletion in the L23 signalling loop [20] has very little effect on bypassing ( Fig. 2d ). Deletion of the L22 loop consisting of residues 84–97, which forms part of the constriction, reduced bypassing by 50%. Additional deletions of constriction site residues in L4 (residues 63–64), did not have any further effect ( Fig. 2d ). The effect of one large deletion from L22 (Δ84–97) on bypassing may be explained by assuming that this deletion removed (part of) the potential interaction partner for the critical residues in the 14–30 region of gp60. Thus, L22 may constitute one of the contacts; however, further interaction partners (for example, 23S rRNA) may be involved. Putative elements upstream of the take-off site Next, we asked whether the mRNA region following nt 90 (after codon 30) but preceding the SL element in the 5′ part of the gap region (nt 91–138) affects bypassing. Prediction of the mRNA structure using mfold and the results of chemical probing [10] suggested the existence of a SL structure upstream of the gap ( Fig. 3a ; Supplementary Fig. 2a,b ). Introducing two synonymous replacements in the upper part of the putative SL (2M) or four synonymous replacements (4M) that should disrupt the SL essentially abolished bypassing ( Fig. 3b ), which suggested a critical role of the mRNA sequence upstream of the gap. Introducing compensatory mutations, which were expected to restore the secondary structure of the upper part (2MC), did not restore bypassing, whereas compensatory mutations for the whole SL (4MC) resulted in partial rescue. The latter observation suggests that the secondary structure of the lower part of the region is important. Why compensatory mutations in the upper part did not restore bypassing is more difficult to explain. One reason may be that the mutations induced formation of an alternative secondary structure, which did not support bypassing. It is also possible that the secondary structure of the region upstream of the gap is different in solution and on the ribosome, such that ‘compensatory’ mutations in the upper part of the SL do not restore the secondary structure. Alternatively, a specific sequence in the region may be important, for example, for interactions with the ribosome. A structure of the mRNA bound to the ribosome during bypassing would be required to distinguish between these possibilities. 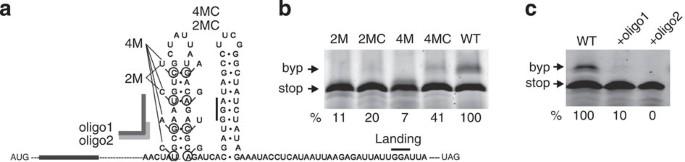Figure 3: The mRNA sequence upstream of the take-off site. (a) Sequence and putative secondary structure of the mRNA upstream of the take-off site predicted by mfold (http://mfold.rna.albany.edu/). Circles indicate mutations (M) introduced to disrupt (2M and 4M) or restore (2MC and 4MC, with C for compensatory) the putative secondary structure. (b) Bypassing with 2M, 2MC, 4M and 4MC mRNA constructs. (c) Bypassing in the presence of DNA oligonucleotides complementary to nucleotides 70–106 (oligo 1) or 70–99 (oligo 2) of gene 60 mRNA (n=6). Figure 3: The mRNA sequence upstream of the take-off site. ( a ) Sequence and putative secondary structure of the mRNA upstream of the take-off site predicted by mfold ( http://mfold.rna.albany.edu/ ). Circles indicate mutations (M) introduced to disrupt (2M and 4M) or restore (2MC and 4MC, with C for compensatory) the putative secondary structure. ( b ) Bypassing with 2M, 2MC, 4M and 4MC mRNA constructs. ( c ) Bypassing in the presence of DNA oligonucleotides complementary to nucleotides 70–106 (oligo 1) or 70–99 (oligo 2) of gene 60 mRNA ( n =6). Full size image We also sought to disrupt putative 5′SL structures by adding two complementary oligonucleotides ( Fig. 3a ). The oligonucleotides did not affect translation as such, because the ribosome can efficiently dissolve duplexes of moderate stability [21] . However, bypassing was abolished ( Fig. 3c ), underscoring the importance of mRNA structure in the region upstream of the gap. The non-coding gap sequence The crucial role for translational bypassing of the SL structure formed by the GGA codon, the stop codons and the 5′ part of the non-coding gap region is well documented [4] , [7] , [8] , [9] , [17] . In comparison, the importance and structure of the 3′ part of the gap are less clear. We varied the length of the 3′ gap by deleting 6 or 12 nt or inserting up to seven copies of the unstructured 6-nt CUCAUA cassette, which extended the 3′ gap region by 6 to 42 nt; in these experiments the SD-like sequence GAG remained at its original distance from the landing GGA codon ( Fig. 4a ). Shortening the 3′ gap increased bypassing, whereas increasing the length of the gap reduced bypassing ( Fig. 4b ), and the yield of byp decreased monotonously with increasing gap length ( Fig. 4c ). Such a dependence can be described by an exponential function ( Y = A × R n ), where Y is the observed bypassing efficiency, n is the gap length in nucleotides, A is the portion of ribosomes initiating bypassing at the take-off site and resuming translation once they reached the landing codon and R is the processivity coefficient, that is, the efficiency of traversing a single nucleotide in the gap. The fit yields A =440±30% and R =0.972±0.001. Given the absolute bypassing efficiency on the WT construct (22%), the fraction of the ribosomes that take part in take-off and landing (provided they reached the landing codon) is close to one (440% × 0.22). This suggests that all ribosomes that initiated bypassing continued translation after landing, and R =0.972. This implies that at each step >97% of ribosomes moved forwards, whereas only <3% dissociated from the track or lost their peptidyl-tRNA 2 Gly . The uniformity of sliding suggests that ribosomes traversing the gap are not affected by pausing because of mRNA secondary structures or other potential stalling interactions with the mRNA, such as attempts of codon reading. 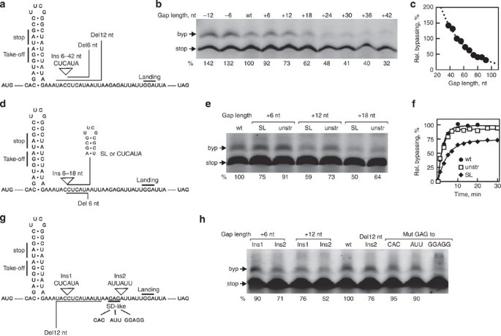Figure 4: Variations in the coding gap. (a) Sequence of the coding gap region. Arrowheads indicate the position where the (CUCAUA)ncassette (1≤n≤7) was inserted (Ins6-42 nt). Deletions of 6 or 12 nucleotides between the SL structure and potential SD-like GAG in the non-structured region are indicated (Del6 nt and Del12 nt). (b) Effect of insertions and deletions in the gap sequence. Changes introduced into the gap sequence are indicated on top, the bypassing efficiency relative to the WT construct at the bottom. (c) Bypassing efficiency as a function of the gap length. Smooth line represents the results of exponential fitting (see text). (d) Introducing structures in the gap. The CUCAUA sequence was deleted (Del 6 nt) and replaced by either a 12-nt step-loop structure (SL; in one, two or three copies) or by an unstructured CUCAUA sequence of the same length as the respective SL constructs (Ins 6-18). (e) Changes in bypassing by increasing the gap length by 6 (+6 nt), 12 (+12 nt) or 18 (+18 nt) nucleotides; the inserted fragment contained either an SL element or a presumably unstructured CUCAUA repeats (unstr) as indicated. The bypassing efficiency with the WT construct was set to 100%. (f) Time courses of synthesis of the bypassing product with the WT mRNA (circles), and mRNAs (+6 nt) containing an additional CUCAUA sequence (open squares) or a SL structure (diamonds). (g) Insertions upstream (Ins1) or downstream (Ins2) of the SD-like GAG codon and the replacements of GAG to CAC, AUU (weak SD sequences) or GGAGG (strong SD sequence). To change the position of the GAG sequence relative to the landing codon, 12 nt were deleted where indicated and inserted at position of Ins2 (Del12/Ins2). (h) Bypassing on mRNAs with mutations in the SD-like sequence (n=8). Figure 4: Variations in the coding gap. ( a ) Sequence of the coding gap region. Arrowheads indicate the position where the (CUCAUA) n cassette (1≤ n ≤7) was inserted (Ins6-42 nt). Deletions of 6 or 12 nucleotides between the SL structure and potential SD-like GAG in the non-structured region are indicated (Del6 nt and Del12 nt). ( b ) Effect of insertions and deletions in the gap sequence. Changes introduced into the gap sequence are indicated on top, the bypassing efficiency relative to the WT construct at the bottom. ( c ) Bypassing efficiency as a function of the gap length. Smooth line represents the results of exponential fitting (see text). ( d ) Introducing structures in the gap. The CUCAUA sequence was deleted (Del 6 nt) and replaced by either a 12-nt step-loop structure (SL; in one, two or three copies) or by an unstructured CUCAUA sequence of the same length as the respective SL constructs (Ins 6-18). ( e ) Changes in bypassing by increasing the gap length by 6 (+6 nt), 12 (+12 nt) or 18 (+18 nt) nucleotides; the inserted fragment contained either an SL element or a presumably unstructured CUCAUA repeats (unstr) as indicated. The bypassing efficiency with the WT construct was set to 100%. ( f ) Time courses of synthesis of the bypassing product with the WT mRNA (circles), and mRNAs (+6 nt) containing an additional CUCAUA sequence (open squares) or a SL structure (diamonds). ( g ) Insertions upstream (Ins1) or downstream (Ins2) of the SD-like GAG codon and the replacements of GAG to CAC, AUU (weak SD sequences) or GGAGG (strong SD sequence). To change the position of the GAG sequence relative to the landing codon, 12 nt were deleted where indicated and inserted at position of Ins2 (Del12/Ins2). ( h ) Bypassing on mRNAs with mutations in the SD-like sequence ( n =8). Full size image We also tested whether inserting of defined SL structures into the 3′ part of the gap affected bypassing. Six nucleotides (CUCAUA) were deleted as shown in Fig. 4a (Del6) and instead a 12-nt SL was inserted in one, two or three copies (SL +6 nt, +12 nt and +18 nt, respectively; Fig. 4d ). For comparison, analogous constructs were made with unstructured sequences (unstr) by inserting a CUCAUA cassette. Introducing a SL motif in up to three copies had a moderate inhibitory effect ( Fig. 4e ). Assuming that all ribosomes could take-off and land (which appears a reasonable assumption, because take-off and landing sites were not altered), the average processivity coefficient was R =0.969 for the mRNAs containing three copies of the SL motif, compared with 0.972 for the unstructured constructs. With the WT mRNA and the +6 nt mRNA construct containing an unstructured CUCAUA sequence, time courses of gp60 synthesis were identical, with half-life time τ 1/2 =2.5 min ( Fig. 4f ). In the presence of the SL structure in the gap, this half-life time increased to τ 1/2 =5 min, suggesting that structures in the 3′ part of the gap slow down the appearance of the byp. Furthermore, we examined whether the position of the SD-like codon GAG affects bypassing. The insertion of a CUCAUA sequence in one or two copies upstream of the GAG, duplication of an unstructured sequence AUUAUU downstream of GAG or deletion of 12 nt (CUCAUA) preceding the GAG codon had a moderate effect, which did not exceed 50%, suggesting that the positioning of the GAG sequence relative to the landing site is not crucial ( Fig. 4h ). Replacements of GAG with CAC or AUU sequences, which cannot engage in SD–aSD (anti-Shine Dalgarno) interactions, had essentially no effect on bypassing, whereas introducing a strong SD sequence, GGAGG, resulted in the synthesis of alternative, longer products. The latter products may result from landing on the two additional GGA codons that are introduced with the enhanced SD sequence [9] . Bypassing signals downstream of the landing site Previous work indicated that replacing the gene 60 sequence following the landing site by reporter constructs did not abolish bypassing [4] , [22] . On the other hand, the bypassing efficiency on truncated gene 60 mRNA in cell lysates was strongly diminished [10] . To assess the minimum length required for bypassing, we tested several mRNA constructs that were truncated at different positions downstream of the landing codon ( Fig. 5a ). The shortest construct that was efficient in bypassing contained 69 nt following the landing site ( Fig. 5b ) and included the whole length of a potential secondary structure element (3′SL) predicted by computational analysis (mfold) and chemical probing [10] . Translation of the T0 control mRNA, which had the same overall length as the WT construct but contained a stop codon at the indicated position ( Fig. 5a ), resulted in formation of a peptide distinct from the stop product ( Fig. 5b ), which shows that the difference in the size between the stop product and of the shortest expected byp from the T1 construct should have been sufficient to resolve the two translation products on the gel. 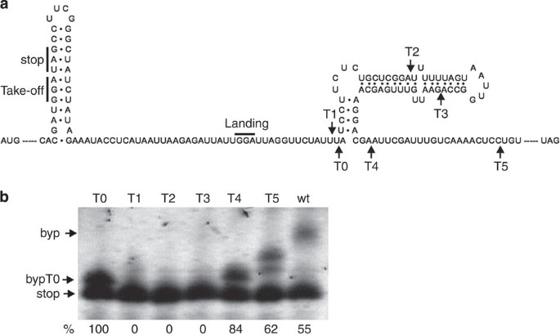Figure 5: Assessment of the minimum mRNA length required for bypassing. (a) Sequence and putative secondary structure of the downstream part of mRNA. Positions of mRNA truncations (Truncations T1–T5) are indicated by arrows. T0, control construct of the same length as the parent mRNA (WT), but with a stop codon after the landing site preceding the putative downstream mRNA structured element. (b) Bypassing efficiency with the truncated mRNA constructs (n=2). Figure 5: Assessment of the minimum mRNA length required for bypassing. ( a ) Sequence and putative secondary structure of the downstream part of mRNA. Positions of mRNA truncations (Truncations T1–T5) are indicated by arrows. T0, control construct of the same length as the parent mRNA (WT), but with a stop codon after the landing site preceding the putative downstream mRNA structured element. ( b ) Bypassing efficiency with the truncated mRNA constructs ( n =2). Full size image Next, we tested which features of the 3′SL structure are essential ( Fig. 6a ). A single G-to-C mutation 64 nt downstream of the landing codon, which is expected to weaken the lower stem of the 3′SL, reduced the bypassing efficiency by 50% ( Fig. 6b ). Deletion of a 6-nt GGUUCU sequence four nucleotides after the landing site (Del1) did not diminish bypassing ( Fig. 6c ); however, additional translation products appeared, suggesting that the fidelity of landing was compromised. In contrast, insertion of a CCGCCG sequence 3 nt downstream of the landing site (Ins1), deletion of a part of the putative secondary structure element (Del 2) or a single U to AA mutation that is expected to distort the local mRNA structure (Mut2) all abolished bypassing ( Fig. 6c ). Surprisingly, removing the putative secondary structure element (Del3) or inserting the same sequence in reverse direction (Rev1) had almost no effect ( Fig. 6d ). Although a 3′SL element probably can form even when the sequence is reversed (Rev1), efficient bypassing in the absence of the presumed 3′SL structure (Del3) can only be explained by the formation of alternative mRNA structures. Mfold predictions suggested that Del3 mRNA may form an alternative secondary structure, which is only four nucleotides closer to the landing codon ( Supplementary Fig. 2c ), which does not abolish bypassing (see Del1). In contrast, Mut2 and Del2 mutations appear to disfavour the WT 3′SL structure and may form alternative helices, which are further away from the landing site ( Supplementary Fig. 2d ). By analogy with the Ins1 mutant, such a shift in the position of the putative helix should abolish bypassing. Thus, efficient bypassing may depend on the presence of a secondary structure element within a particular distance from the landing site. 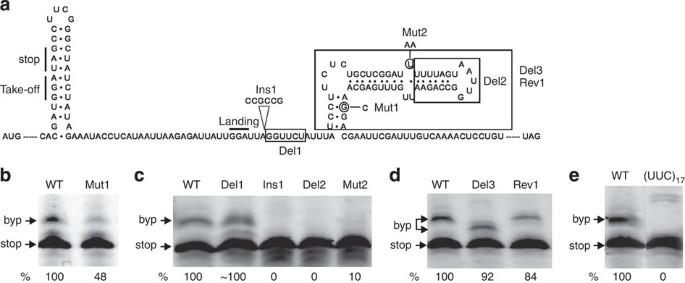Figure 6: Structure requirements for the mRNA region downstream the landing codon. (a) Sequence and putative secondary structure of the region downstream the landing site (from mfold). Positions of mutations (Mut1 and Mut2), deletions (Del1 and Del2) and insertion (Ins1) are indicated. (b) Effect of a single G to C replacement 65 nt downstream of the landing codon. (c) Effects of deletions, insertions and mutations in the 3′SL. (d) Deletion of the putative mRNA secondary structure element (Del3) or insertion of the same element in a reverse direction (Rev1). (e) Replacement of the mRNA sequence downstream of the landing codon by a poly(UUC)17sequence. Efficiency of translational bypassing with the WT mRNA construct was set to 100% (n=8). Figure 6: Structure requirements for the mRNA region downstream the landing codon. ( a ) Sequence and putative secondary structure of the region downstream the landing site (from mfold). Positions of mutations (Mut1 and Mut2), deletions (Del1 and Del2) and insertion (Ins1) are indicated. ( b ) Effect of a single G to C replacement 65 nt downstream of the landing codon. ( c ) Effects of deletions, insertions and mutations in the 3′SL. ( d ) Deletion of the putative mRNA secondary structure element (Del3) or insertion of the same element in a reverse direction (Rev1). ( e ) Replacement of the mRNA sequence downstream of the landing codon by a poly(UUC) 17 sequence. Efficiency of translational bypassing with the WT mRNA construct was set to 100% ( n =8). Full size image To further test the importance of secondary structure, we replaced the mRNA sequence following the landing codon by an unstructured stretch consisting of 17 UUC repeats ((UUC) 17 ). With that mRNA, no byp of the expected length was observed. Instead, some long, low-abundance peptides appeared, which may stem from incorrect landing at the glycine codons preceding the landing codon. These results suggest that the mRNA region downstream of the coding gap is important for bypassing and that secondary structure formation is crucial. However, there is no stringent requirement for one particular structure of the 3′SL, as different alternative secondary structures appear to support bypassing. The present experiments recapitulate translational bypassing in a fully reconstituted translation system consisting of purified ribosomes, translation factors and aminoacyl-tRNAs. Our results indicate that all major determinants for bypassing are specified by the gene 60 mRNA itself and the efficiency of synthesis of the full-length product depends on the interplay between signals in the mRNA and the ability of the ribosome to slide over the coding gap in a processive way. We found that the nascent peptide and the mRNA structure upstream of the gap region (5′SL) and downstream of the landing site (3′SL) have an important role ( Fig. 7 ). Mutations of any of these elements led to a strong reduction in the bypassing efficiency. The relative contributions of each of these elements in vivo may vary, depending on genetic background [22] and changes in the mRNA or tRNA 2 Gly (refs 4 , 9 , 11 , 17 , 23 ) or on the ribosome elements that are known to affect bypassing, such as protein L9 (refs 11 , 14 ). 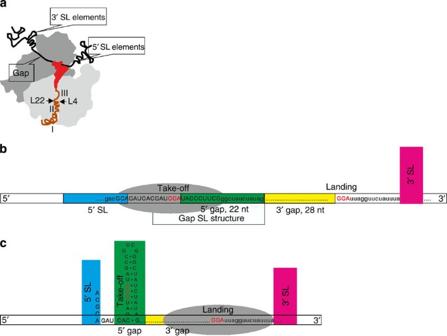Figure 7: mRNA-encoded signals for translational bypassing in T4gene 60mRNA. (a) Schematic of the ribosome with putative mRNA secondary structures upstream of the gap (5′SL), the gap region and putative structures downstream the gap (3′SL) at the moment when bypassing is initiated. Peptidyl-tRNA2Glyis shown in red. The nascent peptide (46 amino acids, brown) can be divided into three regions. Amino acids 1–13 (region I) may anchor the nascent peptide to the surface of the ribosome. Amino acids 14–30 (region II) are located within the exit tunnel after the constriction formed by ribosomal proteins L4 and L22; amino acids on one side of the putative peptide helix within the tunnel have a strong effect on bypassing. Amino acids 31–47 (region III) reside in the cavity between the peptidyl transferase region and the L4–L22 constriction. The 30S and 50S ribosomal subunits are shown in dark and light grey, respectively. (b) The position of the ribosome (grey oval) at the onset of bypassing. 5′SL and 3′SL structures are shown in blue and red, respectively, the 5′ and 3′ parts of the gap sequence are green and yellow, respectively. A large part of the 5′SL, and the SL part of the gap are unfolded (indicated by horizontal bars) and reside in the mRNA channel of the ribosome. The 3′ part of the gap region is predominantly unfolded as well (horizontal bar), whereas the 3′SL element is structured10(vertical bar). (c) Upon movement of the ribosome onto the landing site, the 5′SL upstream of the gap and the 5′SL in the gap refold (vertical bar), whereas the ribosome covers most of the unstructured 3′ part of the gap up to the presumably structured 3′SL (vertical bar). Figure 7: mRNA-encoded signals for translational bypassing in T4 gene 60 mRNA. ( a ) Schematic of the ribosome with putative mRNA secondary structures upstream of the gap (5′SL), the gap region and putative structures downstream the gap (3′SL) at the moment when bypassing is initiated. Peptidyl-tRNA 2 Gly is shown in red. The nascent peptide (46 amino acids, brown) can be divided into three regions. Amino acids 1–13 (region I) may anchor the nascent peptide to the surface of the ribosome. Amino acids 14–30 (region II) are located within the exit tunnel after the constriction formed by ribosomal proteins L4 and L22; amino acids on one side of the putative peptide helix within the tunnel have a strong effect on bypassing. Amino acids 31–47 (region III) reside in the cavity between the peptidyl transferase region and the L4–L22 constriction. The 30S and 50S ribosomal subunits are shown in dark and light grey, respectively. ( b ) The position of the ribosome (grey oval) at the onset of bypassing. 5′SL and 3′SL structures are shown in blue and red, respectively, the 5′ and 3′ parts of the gap sequence are green and yellow, respectively. A large part of the 5′SL, and the SL part of the gap are unfolded (indicated by horizontal bars) and reside in the mRNA channel of the ribosome. The 3′ part of the gap region is predominantly unfolded as well (horizontal bar), whereas the 3′SL element is structured [10] (vertical bar). ( c ) Upon movement of the ribosome onto the landing site, the 5′SL upstream of the gap and the 5′SL in the gap refold (vertical bar), whereas the ribosome covers most of the unstructured 3′ part of the gap up to the presumably structured 3′SL (vertical bar). Full size image Our data suggest the following mechanism of translational bypassing ( Fig. 7 ). When translating the 5′ ORF up to the take-off GGA codon, the ribosome has to unwind the 5′SL upstream of the gap and the SL element in the 5′ part of the gap region. With the take-off GGA in the P site, the whole length of the 5′gap SL and a large part of the downstream 5′SL are probably occluded in the mRNA-binding tunnel of the ribosome, and peptidyl-tRNA 2 Gly is bound in the P site. For the mRNA to become mobile, the codon–anticodon duplex must be disrupted. This may be brought about by a conformational rearrangement of the ribosome, for example, the formation of a highly rotated chimeric intermediate similar to that formed during EF-G-catalysed translocation [24] , [25] , [26] or frameshifting [27] . Although the codon–anticodon interactions are weakened, the retention of peptidyl-tRNA Gly in the ribosome is ensured by the interactions of the nascent peptide with the ribosome, presumably through both unspecific anchoring of the N-terminal part of gp60 emerging from the ribosome peptide exit tunnel and specific interactions of the part of nascent peptide residing in the exit tunnel. Ribosome sliding over the gap is uniformly processive and rapid. The high speed and processivity of sliding is consistent with the idea that the ribosome does not systematically scan the codons in the gap [9] , as scanning would require multiple attempts of forming codon–anticodon interactions in the P site, which—judging from codon recognition in the P site during initiation—is a relatively slow process [28] . Our data suggest that efficient landing requires that the mRNA downstream of the landing site is structured. Presumably, the 3′SL stalls the ribosome, thereby facilitating the landing. At the same time, the 5′SL in the coding part of the mRNA and the SL element in the 5′ part of the gap leave the ribosomal mRNA tunnel and may re-fold, thereby preventing backward sliding of the ribosome ( Fig. 7 ). The exact role of the 5′SL upstream of the gap region is not known. We speculate that it may help to maintain the directionality of ribosome gliding over the gap by re-forming the 5′SL as soon as the ribosome vacates the respective mRNA stretch. The 5′SL may also help re-folding or maintaining the SL in the 5′ part of the gap, which is essential for bypassing. The 5′SL alone or in combination with the SL element in the 5′ gap may interact with protein L9, thereby contributing to the processivity of sliding or the fidelity of landing codon selection. Finally, it may affect the function of L1, the protein which influences the retention of tRNA [29] and the formation of a particular, over-rotated conformation of the ribosome [27] . Previous in-vivo experiments did not implicate the region immediately upstream the gap in the mechanism of bypassing either because the effect of specific mutations was not tested directly or because in vivo the effect is mimicked by contributions of other elements, which are more important under in-vivo conditions. In this context, we note an as yet unexplained effect on bypassing of sequences at the ribosome-binding site 5′ to the start codon [22] , which was interpreted in terms of a potential influence of neighbouring ribosomes in a polysome. The 5′SL may take over this role on the leading ribosome or when the density of ribosomes on the gene60 mRNA is low. The role of the 3′SL downstream the gap is puzzling. Our present experiments and recent in-vitro translation experiments performed in S30 extracts [10] showed that essentially no byp was observed with mRNAs that were truncated shortly after the coding gap. These findings appear to contradict previous results obtained using different reporters in vivo , which suggested that translational bypassing was observed even when the sequence beyond the fifth nucleotide after the landing codon was replaced by the reporter sequence [4] . Also in our translation system, the deletion of nt 264–316 in the 3′ region did not affect bypassing when the remaining mRNA sequence was present. One possible explanation for these observations is that the bypassing signals in the 3′ coding region are not sequence-specific and can be provided by different mRNA sequences, which expose an mRNA hairpin located at a particular distance from the landing codon. A steric hindrance provided by the secondary structure element may stimulate landing, although further experiments will be required to confirm this model. The present data provide the first insight into the kinetic mechanism of translational bypassing. Synthesis of the peptide up to the take-off glycine (47 amino acids) is completed within less than 1 min (not shown). We did not observe a prolonged pausing at the UAG stop codon, which may explain why under normal conditions the efficiency of bypassing is not defined by the competition between termination and take-off, although at elevated concentrations release factor 1 can reach the UAG codon and termination can compete with bypassing [8] . The efficiencies of both take-off and landing (for those ribosomes that reached the landing site) are close to 1 ( Fig. 4 ). However, a part of the ribosomes (and/or tRNA) may be lost from the mRNA track during sliding. At any time, >97% of ribosomes successfully move by one nucleotide towards the landing site, whereas <3% are lost due to drop-off. The loss of a small portion of active sliding complexes at each nucleotide step explains why the bypassing efficiency decreases with increasing gap length. From the length of the gp60 fragment synthesized in the present experiments (90 amino acids), and the half-time of synthesis (150 s), the estimated average translation rate of the byp is about 0.6 amino acid/s. The average translation rate is not altered when the gap length is increased by insertion of a non-structured sequence element ( Fig. 4h ). This suggests that the time required for traversing the gap is small compared with the time required for the synthesis of the peptide. In contrast, when a short SL structure was inserted, the average rate of synthesis decreased to 0.3 amino acid/s. Thus, even a thermodynamically weak SL structure (Δ G ° of the inserted helix is −5 kcal mol −1 , as calculated by mfold) significantly retards the movement through the gap, thereby affecting the overall synthesis rate. Despite the kinetic effect, inserting a defined SL structure in the 3′ gap part reduced the bypassing efficiency by only 15%. Similarly, chemical probing suggest that the 3′ end is predominantly unstructured in solution, and weak potential secondary structure elements that may exist are not important for bypassing [10] . These results argue against the existence of a defined mRNA secondary structure in the 3′ part of the coding gap region, which is spooled into the A site during the movement of the ribosome over the gap. When moving along the mRNA, the ribosome does not recognize alternative GGA codons within the gap [9] . The SD-like sequence has a moderate effect but may be important for the fidelity of landing site selection, particularly in the context of other mutations [8] , [9] , [23] . Taken together with previous genetic work and mRNA structural probing, the present biochemical and mutational analyses provide a detailed insight into the signals for translational bypassing. Nevertheless, crucial details of the mechanism remain obscure, such as why ribosomes start to slide, or whether the conformation of ribosomes changes during bypassing, or the role of protein L9 and the structural dynamics of tRNA 2 Gly . Furthermore, because many different signals contribute, the pathway by which efficient bypassing is stimulated may depend on experimental details, for example, the nature of reporter constructs, expression levels or the presence of mutations. Regardless of the exact kinetic pathway, the existence of efficient bypassing demonstrates how the ribosome–guided by elements specified by the mRNA–is able to overcome the fundamental co-linearity rule of translation. The ability of the ribosome to glide over the mRNA track must have evolved in response to the needs of normal translation. The conformation of the ribosome, which is stabilized during translational bypassing, may represent one of the intermediates during tRNA–mRNA translocation or upon sliding over the mRNA during translation initiation, for example, on mRNAs lacking an SD sequence or on polycistronic mRNAs. Future progress in understanding the kinetics of translational bypassing will show whether the ribosome’s capacity to slide is more commonly used than thought so far and whether it can be utilized for engineering programmed bypassing constructs for the controlled expression of designer proteins. Materials Biochemicals were from Merck, nucleotide triphosphates from Jena Bioscience. The following oligonucleotides were used in the experiment of Fig. 3 : Oligo 1, 5′-CATTCGCATAGTTCATTGAAGAGGATTTAATAGAACG-3′; Oligo2: 5′-ATAGTTCATTGAAGAGGATTTAATAGAACG-3′. [ 3 H]methionine and [ 14 C]leucine were from Hartmann Analytics. Bodipy-FL-succinimidyl ester and Lumio Green Detection Kit were from Invitrogen. Total E. coli tRNA was from Roche and oligonucleotides were from IBA. 70S ribosomes, EF-Tu, EF-G, IF1, IF2, IF3, [ 3 H]Met-tRNA fMet and f[ 3 H]Met-tRNA fMet were prepared from E. coli [30] , [31] , [32] . Site-directed mutagenesis of the WT gene 60 construct [9] was performed using the Quickchange PCR protocol with the appropriate oligonucleotide primers ( Supplementary Table 1 ). mRNAs were produced by T7 RNA-polymerase in-vitro transcription and purified by ion-exchange chromatography on HiTrap Q HP 5 ml column (GE Healthcare). To prepare fluorescence-labelled [ 3 H]Met-tRNA fMet (Bpy-Met-tRNA fMet ), HPLC-purified [ 3 H]Met-tRNA fMet (30 μM) was incubated with BODIPY-FL sulfosuccinimidyl ester (Bpy-SSE; Invitrogen, D6140; 4 mM) in 20 mM HEPES buffer (pH 8.5) for 4 min at 0 °C. The reaction was stopped by adding 0.2 M potassium acetate (pH 5), and the tRNA was precipitated by ethanol. Excess dye was removed by four additional ethanol precipitation steps [33] , [34] . The degree of labelling was >97% according to HPLC analysis on Biosuite 250 HR 30 cm SEC column (Waters). Translation Translation was carried out in buffer A (50 mM Tris–HCl, pH 7.5, 70 mM NH 4 Cl, 30 mM KCl and 7 mM MgCl 2 ) at 37 °C, unless stated otherwise. Initiation complexes were formed by incubating ribosomes (0.5 μM), mRNA (1.5 μM), IF1, IF2 and IF3 (0.75 μM each), GTP (1 mM) and either BPY-[ 3 H]Met-tRNA fMet or initiator f[ 3 H]Met-tRNA fMet (0.75 μM), in buffer A at 37 °C for 30 min. Ternary complex EF-Tu–GTP–aminoacyl-tRNA was prepared by incubating EF-Tu (58 μM) with GTP (1 mM), phosphoenol pyruvate (3 mM) and pyruvate kinase (0.1 mg ml −1 ) for 15 min at 37 °C, then adding purified total aa-tRNA (about 60 μM) and EF-G (1 μM) and incubating for 1 min at 37 °C. In vitro translation was started by mixing initiation ribosomal complexes (0.08 μM) with the ternary complexes (24 μM) total aa-tRNA (containing [ 14 C]Leu-tRNA Leu ) and incubated at 37 °C. Reactions were terminated by either shock-freezing aliquots in liquid nitrogen or by adding 2 × loading buffer for SDS–polyacrylamide gel electrophoresis. Samples were treated with RNase A for 30 min and the translation products were separated by Tris-Tricine gel electrophoresis [35] , [36] . Fluorescent and radioactive peptides were detected after gel electrophoresis using FLA-7000 scanner (FujiFilm) and quantified using the Multi-Gauge software. Unless stated otherwise, bypassing efficiency was calculated as the intensity of the N-terminal Bpy label in the byp divided by the sum of intensities from bypassing (byp) and truncated (stop) gp60 bands. Similarly, the efficiency of read-through ( Fig. 1e ) was calculated from the Bpy signal in the read-through band (rt) divided by the sum of intensities of byp, stop and rt bands. When [ 14 C]Leu was used to visualize the byp and stop products ( Fig. 1d ), bypassing efficiency was calculated in the same way, taking into account that the byp product contains five times as many Leu residues as the stop product. To calculate bypassing efficiency from Lumio detection, the intensities of the byp and Δgap products were compared ( Fig. 1c ). Statistics The s.d. were analysed from a large collection of technical and biological replicates. The magnitude of standard deviation depended on the band efficiency: when the bypassing efficiency was low, <10%, the standard deviation was about 30% of the given value, for example, 10±3%. For the higher bypassing efficiencies, standard deviation was lower, about 10%, for example, absolute bypassing efficiency for the WT construct at standard conditions was 22±2%. How to cite this article: Samatova, E. et al. High-efficiency translational bypassing of non-coding nucleotides specified by mRNA structure and nascent peptide. Nat. Commun. 5:4459 doi: 10.1038/ncomms5459 (2014).